The bacterial tubulin FtsZ requires its intrinsically disordered linker to direct robust cell wall construction The bacterial GTPase FtsZ forms a cytokinetic ring at midcell, recruits the division machinery and orchestrates membrane and peptidoglycan cell wall invagination. However, the mechanism for FtsZ regulation of peptidoglycan metabolism is unknown. The FtsZ GTPase domain is separated from its membrane-anchoring C-terminal conserved (CTC) peptide by a disordered C-terminal linker (CTL). Here we investigate CTL function in Caulobacter crescentus . Strikingly, production of FtsZ lacking the CTL (ΔCTL) is lethal: cells become filamentous, form envelope bulges and lyse, resembling treatment with β-lactam antibiotics. This phenotype is produced by FtsZ polymers bearing the CTC and a CTL shorter than 14 residues. Peptidoglycan synthesis still occurs downstream of ΔCTL; however, cells expressing ΔCTL exhibit reduced peptidoglycan crosslinking and longer glycan strands than wild type. Importantly, midcell proteins are still recruited to sites of ΔCTL assembly. We propose that FtsZ regulates peptidoglycan metabolism through a CTL-dependent mechanism that extends beyond simple protein recruitment. Cell shape in bacteria is maintained by the peptidoglycan (PG) cell wall, a covalently linked network of glycan strands crosslinked by short peptides that provides mechanical integrity to the envelope and prevents cell lysis in the face of turgor pressure [1] . During growth and division, PG is remodelled by synthetic and hydrolytic enzymes whose activities must be precisely coordinated to preserve the integrity of the cell wall. Moreover, achieving specific cell shapes and forming new cell poles during division requires that PG remodelling be spatially organized. The cytoskeletal proteins FtsZ and MreB are dynamically associated with and direct localization of cell wall remodelling enzymes during cell division and elongation [1] , [2] . In addition, polymers of FtsZ, MreB and the intermediate filament-like protein, crescentin, have been implicated in the mechanical regulation of cell shape [2] , [3] , [4] , [5] . However, it is unclear how the biochemical and biophysical properties of these cytoplasmic membrane-associated proteins influence PG remodelling in the periplasm to define the shape of the cell [1] , [2] . FtsZ polymerizes at midcell to form the Z-ring, a dynamic structure on which the cell division machinery (divisome) assembles [6] . The divisome comprises dozens of proteins including factors that regulate FtsZ structure and membrane attachment, remodel the cell wall and invaginate the membranes. In most bacteria, FtsZ is the first protein to arrive at the incipient division site, and it is required for recruitment of cell wall regulators and divisome proteins, which occurs in serial stages [7] , [8] , [9] . In addition to its primary role in cell division, in at least some organisms, FtsZ directs PG synthesis for elongation of the cell before cell envelope constriction [10] , [11] . Apart from regulating PG remodelling and envelope invagination through protein recruitment, in vitro studies suggest that FtsZ is capable of generating force and deforming membranes [4] , [12] . On the basis of these findings, a mechanical role for FtsZ in inner membrane constriction has been proposed. However, it is not known whether force generation by FtsZ is required in vivo , nor is it clear how FtsZ-mediated force might be coupled to PG remodelling to coordinately invaginate the multiple layers of the cell envelope during cytokinesis [13] . FtsZ is structurally similar to eukaryotic tubulin [14] , [15] and polymerizes in a GTP-dependent manner, forming linear protofilaments [16] , [17] . The FtsZ monomer can be divided into four regions: (i) a short N-terminal peptide, (ii) a conserved GTPase domain essential for polymerization, (iii) an intrinsically disordered C-terminal linker (CTL) and (iv) a C-terminal conserved peptide (CTC) that interacts with membrane-tethering proteins ( Fig. 1a ) [18] . A comparison of FtsZ across species reveals that the CTL is poorly conserved in sequence, and varies widely in length from ∼ 9 to more than 300 residues. In Escherichia coli and Bacillus subtilis , the CTL was recently demonstrated to be essential for cell division, playing a sequence-independent role in executing cytokinesis [19] , [20] . Almost any intrinsically disordered sequence similar in length to the native CTL was sufficient to support normal cytokinesis, even if there was no detectable sequence similarity to the native CTL. The authors of these studies proposed that the CTL functions as an entropic spring [20] or flexible linker [19] that is crucial for Z-ring formation and constriction. 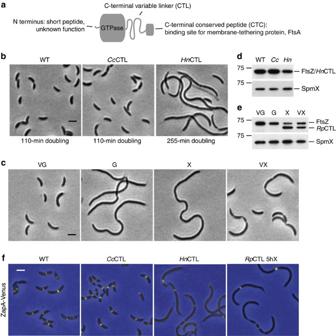Figure 1: TheC. crescentusCTL fulfils an essential, sequence-dependent function. (a) Domain organization of FtsZ. (b) Phase contrast images of strains expressing WT (NA1000),CcCTL control (EG776) orHnCTL (EG769)ftsZ variants as the only copy of FtsZ in the cell and their corresponding doubling times in PYE medium. Scale bar, 2 μm. (c) Phase contrast images of strain EG1060, bearing vanillate (V)-induced expression of WTftsZ and xylose (X)-induced expression ofRpCTLftsZ. Cells were grown in the presence of the indicated inducer or glucose (G) for 5 h before imaging. Scale bar, 2 μm. (d,e) Immunoblots against lysates from strains inb,cusing FtsZ (top) or SpmX antisera (bottom). Owing to lack of a specific antibody raised against a loading control distinct enough in size from FtsZ and each of the variants used in this study, SpmX was probed against identical samples on a separate blot.Cc=CcCTL,Hn=HnCTL. FtsZ antiserum was raised against the entire WT FtsZ molecule. Some of the reduction in signal observed forHnCTL andRpCTL may be attributable to loss of CTL-derived epitopes. Positions of molecular weight markers (kDa) are indicated (left). (f) ZapA-Venus fluorescence (yellow) overlaid on phase contrast (blue) images of cells producing the indicated FtsZ CTL variants and ZapA-Venus. WT (EG941),CcCTL (EG1418) andHnCTL (EG1389) were produced from theftsZlocus as the only FtsZ in the cell.RpCTL (EG1419) production was induced with xylose while depleting WT FtsZ for 5 h before imaging. Scale bar, 2μm. Figure 1: The C. crescentus CTL fulfils an essential, sequence-dependent function. ( a ) Domain organization of FtsZ. ( b ) Phase contrast images of strains expressing WT (NA1000), Cc CTL control (EG776) or Hn CTL (EG769) fts Z variants as the only copy of FtsZ in the cell and their corresponding doubling times in PYE medium. Scale bar, 2 μm. ( c ) Phase contrast images of strain EG1060, bearing vanillate (V)-induced expression of WT fts Z and xylose (X)-induced expression of Rp CTL fts Z. Cells were grown in the presence of the indicated inducer or glucose (G) for 5 h before imaging. Scale bar, 2 μm. ( d , e ) Immunoblots against lysates from strains in b , c using FtsZ (top) or SpmX antisera (bottom). Owing to lack of a specific antibody raised against a loading control distinct enough in size from FtsZ and each of the variants used in this study, SpmX was probed against identical samples on a separate blot. Cc = Cc CTL, Hn = Hn CTL. FtsZ antiserum was raised against the entire WT FtsZ molecule. Some of the reduction in signal observed for Hn CTL and Rp CTL may be attributable to loss of CTL-derived epitopes. Positions of molecular weight markers (kDa) are indicated (left). ( f ) ZapA-Venus fluorescence (yellow) overlaid on phase contrast (blue) images of cells producing the indicated FtsZ CTL variants and ZapA-Venus. WT (EG941), Cc CTL (EG1418) and Hn CTL (EG1389) were produced from the ftsZ locus as the only FtsZ in the cell. Rp CTL (EG1419) production was induced with xylose while depleting WT FtsZ for 5 h before imaging. Scale bar, 2μm. Full size image Here we study FtsZ function in the α-proteobacterium Caulobacter crescentus , which has long been used as a model for investigating cell shape, development and regulation of cell cycle-dependent events such as cytokinesis [21] . Among bacteria, α-proteobacteria stand out as having exceptionally long FtsZ CTLs [18] , [22] . Whereas the CTLs of E. coli and B. subtilis FtsZ are ∼ 50 amino acids long, that of C. crescentus is 172 amino acids, and many α-proteobacteria have CTLs longer than 300 amino acids. In the present work, we set out to understand the physiological significance of the long CTL in C. crescentus FtsZ, and in the process uncovered a surprising requirement for the FtsZ CTL in regulating specific aspects of PG remodelling. From these findings, we propose that FtsZ regulates PG metabolism through a CTL-dependent mechanism that is in addition to its ability to recruit proteins to midcell. The FtsZ CTL fulfils an essential function in C. crescentus To investigate the function of the CTL in C. crescentus , we engineered a panel of C. crescentus FtsZ CTL variants bearing the wild-type (WT) C. crescentus CTL ( Cc CTL), three other α-proteobacterial CTLs (from Hyphomonas neptunium ( Hn CTL), Rickettsia parkeri ( Rp CTL) or Magnetospirillum magneticum ( Mm CTL)), or the much shorter E. coli CTL ( Ec CTL) in place of the C. crescentus CTL ( Table 1 , Supplementary Fig. 1 ). As the primary sequence conservation is low in this region of FtsZ, the most similar CTL we tested, Hn CTL, is only 18% identical and 35% similar to Cc CTL. The other CTLs tested had no detectable sequence similarity ( Supplementary Fig. 1 ). Using allele exchange, we asked whether any of these variants could replace WT ftsZ and found that only Cc CTL or Hn CTL yielded viable C. crescentus cells ( Table 1 ). Moreover, while the control Cc CTL strain was morphologically indistinguishable from WT and grew at a similar rate, Hn CTL cells were filamentous and slow growing ( Fig. 1b ). Table 1 CTL variants used in this study. Full size table To examine the phenotypes of cells producing noncomplementing FtsZ CTL variants, we created strains in which the vanillate-inducible promoter (P vanA ) drives expression of the only copy of WT ftsZ and the xylose-inducible promoter (P xylX ) drives expression of a CTL variant ( Supplementary Fig. 2a ). Expressing WT ftsZ from either promoter using this strategy supports normal cytokinesis ( Supplementary Fig. 2b,c ). When Rp CTL, Mm CTL or Ec CTL was produced while depleting WT FtsZ, cells became filamentous, consistent with their inability to complement loss of ftsZ ( Fig. 1c , Supplementary Fig. 2d ). We examined steady-state levels of each variant by immunoblotting. While Rp CTL and Hn CTL proteins were detected at near-WT levels, Mm CTL and Ec CTL were undetectable ( Fig. 1d,e , Supplementary Fig. 2e ). WT FtsZ was depleted to 10–40% of normal levels in the absence of vanillate after 6.5 h ( Fig. 1e , Supplementary Fig. 2c,e ). We assessed Z-ring formation in cells producing WT FtsZ, Cc CTL, Hn CTL or Rp CTL by imaging a fluorescent fusion of the FtsZ-binding protein (ZBP), ZapA ( Fig. 1f ). ZapA-Venus localized to midcell bands or rings in each. However, in Hn CTL-producing cells, patches of ZapA-Venus were also observed, suggesting a reduced capacity to form Z-rings. Length is not the primary determinant of CTL function To further decipher the essential regions of the CTL, we asked whether FtsZ variants lacking portions of the Cc CTL support cytokinesis. We engineered CTL variants bearing only the N-terminal 34, 68, 102 or 136 residues (Nt34, Nt68, Nt102 and Nt136) or C-terminal 36, 70, 104 or 138 residues (Ct36, Ct70, Ct104 and Ct138) of the CTL ( Fig. 2a ). Surprisingly, most of these variants supported viability when expressed as the only copy of ftsZ ( Fig. 2b,d ). However, while the first 34 residues of the CTL were dispensable for full function ( Fig. 2b , Ct138), all other deletion variants were filamentous. The two shortest variants tested contained only 34 or 36 residues yet supported cytokinesis, suggesting that C. crescentus tolerates large changes to CTL length while maintaining viability. Interestingly, two variants of intermediate length (Ct70 and Nt102) were nonfunctional and yielded filamentous cells when produced while depleting WT FtsZ ( Fig. 2c,e ). These data indicate that length is not the primary determinant of CTL function in C. crescentus , as the noncomplementing variants are almost identical in length to two complementing variants. Similarly, Ct138 and Nt136 are almost identical in length; however, Nt136-producing cells are filamentous while Ct138-producing cells divide normally ( Fig. 2b ). 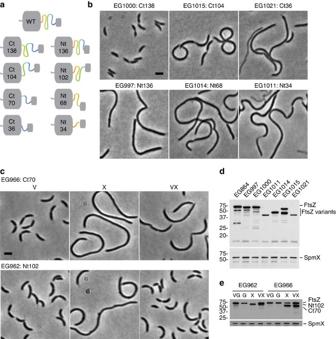Figure 2:C. crescentustolerates large changes to the length of the CTL. (a) Graphical representation of the CTL deletion variants analysed. Ct138=FtsZ with only the C-terminal 138 residues of the CTL, Nt136=FtsZ with only the N-terminal 136 residues of the CTL and so forth. (b) Phase contrast images of strains producing the indicated CTL variants as the only copy of FtsZ in the cell, expressed from theftsZlocus. Scale bar, 2 μm. (c) Phase contrast images of the indicated strains, grown with vanillate (V), xylose (X) or both (VX) for 5 h before imaging. Scale bar, 2 μm. (d,e) Immunoblots against lysates from strains inb,cusing FtsZ (top) or SpmX (bottom) antisera. Positions of molecular weight markers (kDa) are indicated (left). Figure 2: C. crescentus tolerates large changes to the length of the CTL. ( a ) Graphical representation of the CTL deletion variants analysed. Ct138=FtsZ with only the C-terminal 138 residues of the CTL, Nt136=FtsZ with only the N-terminal 136 residues of the CTL and so forth. ( b ) Phase contrast images of strains producing the indicated CTL variants as the only copy of FtsZ in the cell, expressed from the ftsZ locus. Scale bar, 2 μm. ( c ) Phase contrast images of the indicated strains, grown with vanillate (V), xylose (X) or both (VX) for 5 h before imaging. Scale bar, 2 μm. ( d , e ) Immunoblots against lysates from strains in b , c using FtsZ (top) or SpmX (bottom) antisera. Positions of molecular weight markers (kDa) are indicated (left). Full size image The Nt34 and Ct36 variants were both present at low steady-state protein levels ( Fig. 2d ), suggesting that composition of the CTL contributes to FtsZ levels. As proteolysis of FtsZ is a known point of regulation in C. crescentus [23] , [24] , we determined the half-lives of the Hn CTL, Ct138, Nt34 and Ct36 variants and found that, indeed, Nt34 ( t 1/2 = ∼ 27 min) and Ct36 ( t 1/2 = ∼ 23 min) turned over substantially faster than WT FtsZ ( t 1/2 = ∼ 48 min; Supplementary Fig. 2f ). Collectively, the above analyses indicate that the CTL in C. crescentus plays an essential, sequence-dependent role in cell division. Moreover, CTL composition contributes to post-transcriptional regulation of FtsZ levels, including affecting protein turnover. FtsZ lacking the CTL induces bulging and rapid cell lysis Having established that the CTL plays an important role in C. crescentus FtsZ function, we next examined the effects of producing FtsZ completely lacking the CTL (ΔCTL). To do this, we generated a strain bearing vanillate-induced WT ftsZ and xylose-induced ΔCTL . Unexpectedly, induction of ΔCTL caused cells to grow into filaments with localized envelope bulges and to rapidly lyse ( Fig. 3a–c ). In the absence of vanillate, bulges began to appear at 2 h post induction of ΔCTL and were abundant at 4–5 h post induction. Transmission electron microscopy (TEM) of ΔCTL -expressing cells confirmed that most bulges are roughly symmetrical expansions of the cell envelope ( Fig. 3b ). Cells began to lyse by 5 h post induction of ΔCTL ( Fig. 3a,c ). The effects of ΔCTL expression were dominant lethal: bulging and lysis occurred in the presence of vanillate but were delayed when compared with the phenotype in the absence of WT ftsZ induction ( Fig. 3a,c ). Using a second inducible expression system, with P xylX driving expression of ftsZ and the recently described myo-inositol-inducible P iolC (refs 25 , 26 ) driving expression of ΔCTL , we were able to deplete WT FtsZ to <5% of normal levels ( Supplementary Fig. 4a–c ). Bulging and lysis were observed under these conditions as well, indicating that significant amounts of WT FtsZ are not required for the ΔCTL phenotype. ΔCTL expression was also toxic to cells grown in minimal media, causing filamentation, rough cell envelope appearance and lysis ( Supplementary Fig. 4d,e ). Unlike Nt34 or Ct36, deleting the CTL entirely did not have a pronounced effect on FtsZ steady-state protein levels ( Fig. 3d , Supplementary Fig. 4f ). 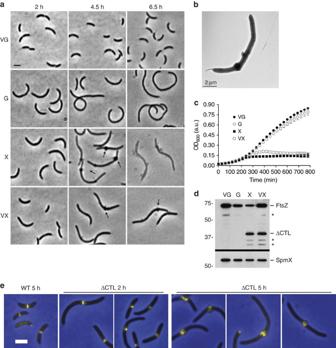Figure 3: ΔCTL production causes dominant lethal envelope bulging and cell lysis. (a) Phase contrast images of cells from strain EG852, with vanillate-induced expression offtsZand xylose-induced expression ofΔCTL. Cells were grown for the indicated amount of time in PYE medium with the indicated inducer (vanillate (V), xylose (X) and/or glucose (G)) before imaging. Arrows highlight envelope bulges. Scale bar, 2 μm. (b) Whole-mount transmission electron micrograph of an EG852 cell grown in PYE xylose for 4 h. (c) Growth of strain EG852 in PYE with the indicated inducers added at time 0, as monitored by OD600. Average±s.d. from three technical replicates is plotted. (d) Immunoblot of lysates from cells inaafter 7 h growth in PYE with the indicated inducers using FtsZ (top) or SpmX antisera (bottom). Asterisks indicate degradation products. Positions of molecular weight markers (kDa) are indicated (left). (e) Merged ZapA-Venus fluorescence (yellow) and phase contrast (blue) images of cells producing WT FtsZ (EG1396) for 5 h or ΔCTL (EG950) for 2 or 5 h. Figure 3: ΔCTL production causes dominant lethal envelope bulging and cell lysis. ( a ) Phase contrast images of cells from strain EG852, with vanillate-induced expression of ftsZ and xylose-induced expression of ΔCTL . Cells were grown for the indicated amount of time in PYE medium with the indicated inducer (vanillate (V), xylose (X) and/or glucose (G)) before imaging. Arrows highlight envelope bulges. Scale bar, 2 μm. ( b ) Whole-mount transmission electron micrograph of an EG852 cell grown in PYE xylose for 4 h. ( c ) Growth of strain EG852 in PYE with the indicated inducers added at time 0, as monitored by OD 600 . Average±s.d. from three technical replicates is plotted. ( d ) Immunoblot of lysates from cells in a after 7 h growth in PYE with the indicated inducers using FtsZ (top) or SpmX antisera (bottom). Asterisks indicate degradation products. Positions of molecular weight markers (kDa) are indicated (left). ( e ) Merged ZapA-Venus fluorescence (yellow) and phase contrast (blue) images of cells producing WT FtsZ (EG1396) for 5 h or ΔCTL (EG950) for 2 or 5 h. Full size image Using ZapA-Venus as a proxy for FtsZ localization, we found that bulges occur at sites of FtsZ assembly ( Fig. 3e ). ZapA-Venus localized to rings in cells producing WT FtsZ, as expected, and localized to the bulges of ΔCTL-producing cells. However, ZapA-Venus localization was more heterogeneous and less focused into a ring in cells producing ΔCTL as compared with WT; this effect was most apparent at 5 h post induction. We verified that ZapA-Venus reported on the localization of FtsZ in each strain by producing an N-terminal CFP fusion to FtsZ or ΔCTL while depleting WT FtsZ ( Supplementary Fig. 4g,h ). Although these fusions were nonfunctional, CFP-FtsZ localized to midcell bands and CFP-ΔCTL was enriched in bulges. Collectively, these data indicate that FtsZ lacking the CTL induces local, toxic effects that lead to loss of envelope integrity and cell lysis. Induction of bulging and lysis is CTL length-dependent All organisms that possess an FtsZ homologue with a CTC bear a CTL of at least approximately nine residues [18] . Moreover, expression of ftsZ lacking the CTL in B. subtilis or another CTL variant in E. coli was reported to cause cell lysis [19] , [20] . This led us to speculate that a minimal CTL might be a conserved requirement to prevent FtsZ-induced cell lysis. To test this, we added residues from the C terminus of the CTL to the ΔCTL variant in single amino-acid increments and examined the effects of expressing these variants while depleting WT FtsZ. Interestingly, we observed an exquisite CTL length dependence for the induction of bulging and lysis ( Fig. 4 ): expression of ftsZ with linkers up to eight amino acids (including four residues introduced by restriction enzyme sites) induced bulging ( Fig. 4a,b ), with a length-dependent decrease in maximum cell width (used as a read-out for envelope bulging; Fig. 4c ). These variants also induced lysis, with the time to lysis increasing with linker length ( Fig. 4d ). FtsZ variants with linkers of 9–12 amino acids did not promote bulging, but induced lysis 6–8 h post induction. Thirteen and fourteen amino-acid linker variants did not induce bulging or rapid lysis, but failed to support cell division. All short-linker variants were produced at similar levels ( Fig. 4b ). 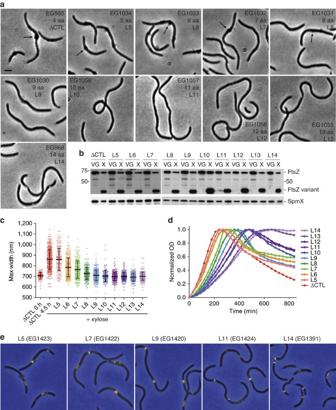Figure 4: Bulging and lysis is CTL length-dependent. (a) Phase contrast images of strains producing FtsZ with the indicated CTL lengths grown with xylose for 4.5 h before imaging. The number of amino acids (aa) in the linker includes four residues added from restriction sites introduced for cloning purposes. Thus, ΔCTL contains a four aa linker. Each strain bears vanillate-inducedftsZand xylose-induced CTL variant. Scale bar, 2 μm. Arrows highlight bulges. (b) Immunoblots of lysates from strains inagrown with vanillate and glucose or with xylose for 6.5 h using FtsZ (top) or SpmX antisera (bottom). Positions of molecular weight markers (kDa) are indicated (left). (c) Maximum widths of cells from strains fromagrown with xylose for 4.5 h and for EG985 grown with vanillate and glucose (ΔCTL VG; expressing WTftsZ). Data points represent the maximum width for each cell in that population. Data are combined from two independent imaging experiments for each strain. ΔCTL X data include two independent experiments with EG985 and one with EG852 (independent, isogenic strains for producing ΔCTL).n=80, 354, 254, 274, 268, 242, 281, 151, 281, 212, 357 and 326 cells for samples as presented from left to right. Line=average width, whiskers=s.d. (d) Growth and lysis of strains froma. Cells were grown with xylose from time 0 and OD was monitored at 600 nm. Final plots were normalized for each data set and represent average data from three technical replicates. The time at which OD began to fall was interpreted as time of initiation of lysis. (e) ZapA-Venus fluorescence (yellow) overlaid on phase contrast (blue) images of cells producing the indicated FtsZ CTL variants and ZapA-Venus. Each variant was induced with xylose while depleting WT FtsZ for 5 h before imaging. Figure 4: Bulging and lysis is CTL length-dependent. ( a ) Phase contrast images of strains producing FtsZ with the indicated CTL lengths grown with xylose for 4.5 h before imaging. The number of amino acids (aa) in the linker includes four residues added from restriction sites introduced for cloning purposes. Thus, ΔCTL contains a four aa linker. Each strain bears vanillate-induced ftsZ and xylose-induced CTL variant. Scale bar, 2 μm. Arrows highlight bulges. ( b ) Immunoblots of lysates from strains in a grown with vanillate and glucose or with xylose for 6.5 h using FtsZ (top) or SpmX antisera (bottom). Positions of molecular weight markers (kDa) are indicated (left). ( c ) Maximum widths of cells from strains from a grown with xylose for 4.5 h and for EG985 grown with vanillate and glucose (ΔCTL VG; expressing WT ftsZ ). Data points represent the maximum width for each cell in that population. Data are combined from two independent imaging experiments for each strain. ΔCTL X data include two independent experiments with EG985 and one with EG852 (independent, isogenic strains for producing ΔCTL). n =80, 354, 254, 274, 268, 242, 281, 151, 281, 212, 357 and 326 cells for samples as presented from left to right. Line=average width, whiskers=s.d. ( d ) Growth and lysis of strains from a . Cells were grown with xylose from time 0 and OD was monitored at 600 nm. Final plots were normalized for each data set and represent average data from three technical replicates. The time at which OD began to fall was interpreted as time of initiation of lysis. ( e ) ZapA-Venus fluorescence (yellow) overlaid on phase contrast (blue) images of cells producing the indicated FtsZ CTL variants and ZapA-Venus. Each variant was induced with xylose while depleting WT FtsZ for 5 h before imaging. Full size image Similar to ΔCTL, we observed patchy, discontinuous ZapA-Venus localization in strains producing short-linker variants that induce early lysis (L5, L7, L9 and L11; Fig. 4e ). In contrast, the L14-producing strain that does not undergo bulging or lysis contained focused Z-rings resembling those found in WT cells. We conclude that a minimal linker of 13–14 amino acids is required to form focused Z-rings and to prevent FtsZ from inducing lethal changes to the cell envelope in C. crescentus . ΔCTL requires the CTC to induce bulging and lysis We next asked whether FtsZ lacking the CTL must be attached to the membrane to invoke its effects. Membrane attachment of FtsZ is mediated by interaction of the CTC with the membrane-tethering protein, FtsA [27] , [28] , [29] ( Fig. 5a ). We therefore generated an FtsZ variant lacking both the CTL and CTC (ΔCTLC). Cells producing ΔCTLC and depleted of FtsZ grew as smooth filaments, similar to cells producing a variant lacking only the CTC (ΔCTC), but did not undergo bulging or rapid lysis ( Fig. 5a–c ), suggesting that membrane attachment is required for ΔCTL to induce its lethal effects. To determine whether the mode of membrane attachment was important, we appended the membrane-targeting sequence (MTS) from E. coli MinD to ΔCTC or ΔCTLC to directly tether these variants to the membrane. Similar to ΔCTLC and ΔCTC, cells producing these constructs (ΔCTC-MTS or ΔCTLC-MTS) grew as smooth filaments that did not rapidly lyse ( Fig. 5a–c ). We conclude that ΔCTL requires the CTC to induce bulging and lysis. As the only known activity of the CTC in C. crescentus is binding to FtsA, our results indicate that membrane attachment by the native membrane anchor is required for the ΔCTL phenotype. 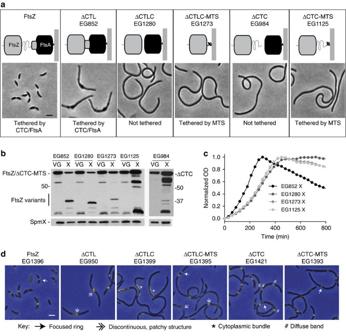Figure 5: ΔCTL requires the membrane-anchoring CTC to invoke bulging and lysis. (a) Schematics and representative phase contrast images of WT cells (FtsZ) and cells producing the indicated FtsZ variants and depleted of WT FtsZ for 5 h. ΔCTLC—FtsZ lacking the CTL and FtsA-binding CTC. MTS—membrane-targeting sequence fromE. coliMinD. ΔCTC—FtsZ lacking the CTC. Scale bar, 2 μm. (b) Immunoblots of lysates from strains inagrown with vanillate and glucose or with xylose for 5 h probed with FtsZ (top) or SpmX antisera. Positions of molecular weight markers (kDa) are indicated. (c) Growth and lysis of strains froma. Cells were grown with xylose from time 0 and OD was monitored at 600 nm. Final plots were normalized for each data set and represent average data from three technical replicates. (d) ZapA-Venus fluorescence (yellow) overlaid on phase contrast (blue) images of cells producing the indicated FtsZ CTL variants and ZapA-Venus. Each variant was induced with xylose while depleting WT FtsZ for 5 h before imaging. Scale bar, 2 μm. Figure 5: ΔCTL requires the membrane-anchoring CTC to invoke bulging and lysis. ( a ) Schematics and representative phase contrast images of WT cells (FtsZ) and cells producing the indicated FtsZ variants and depleted of WT FtsZ for 5 h. ΔCTLC—FtsZ lacking the CTL and FtsA-binding CTC. MTS—membrane-targeting sequence from E. coli MinD. ΔCTC—FtsZ lacking the CTC. Scale bar, 2 μm. ( b ) Immunoblots of lysates from strains in a grown with vanillate and glucose or with xylose for 5 h probed with FtsZ (top) or SpmX antisera. Positions of molecular weight markers (kDa) are indicated. ( c ) Growth and lysis of strains from a . Cells were grown with xylose from time 0 and OD was monitored at 600 nm. Final plots were normalized for each data set and represent average data from three technical replicates. ( d ) ZapA-Venus fluorescence (yellow) overlaid on phase contrast (blue) images of cells producing the indicated FtsZ CTL variants and ZapA-Venus. Each variant was induced with xylose while depleting WT FtsZ for 5 h before imaging. Scale bar, 2 μm. Full size image To determine whether the membrane-targeting variants support Z-ring formation, we examined ZapA-Venus localization in each of the above strains. Although ΔCTC-MTS was nonfunctional, it recruited ZapA-Venus to Z-rings in a manner indistinguishable from WT ( Fig. 5d ). Apparently normal Z-rings were also observed in cells producing ΔCTLC-MTS, although patchy structures like those observed in ΔCTL-producing cells were more prevalent. In cells producing ΔCTLC, ZapA-Venus localized exclusively to cytoplasmic bundles. Eliminating the CTL in conjunction with the CTC was required for formation of these cytoplasmic bundles, as ZapA-Venus localized to diffuse, broad bands in ΔCTC-producing cells. Thus, although targeting to membranes via the CTC is not required for Z-ring formation, the CTC is required for ΔCTL to induce bulging and lysis. Deletion of the CTL may increase FtsZ polymer bundling, an effect that is most apparent in vivo when membrane attachment of ΔCTL is eliminated. ΔCTL must polymerize to induce bulging and lysis Prior work in B. subtilis demonstrated that FtsZ lacking the CTL polymerized poorly [19] and we observed aberrant Z-ring structures in cells producing CTL variants. To address whether C. crescentus ΔCTL has altered polymerization properties, we assessed its self-assembly in vitro . We purified WT FtsZ, ΔCTL and, as a control for effects specific to the ΔCTL phenotype, the L14 short-linker variant that did not induce bulging and lysis but was nonfunctional for cytokinesis. Both ΔCTL and L14 exhibited reduced polymerization when compared with WT, as assessed by high-speed pelleting and right-angle light scattering ( Fig. 6a , Supplementary Fig. 5a ). Correspondingly, the GTPase rates of ΔCTL (1.86±0.04 min −1 (mean±s.e. ), n =3) and L14 (2.89±0.06 min −1 , n =3) were 42 and 65% that of WT FtsZ (4.44±0.10 min −1 , n =3), respectively, at 4 μM ( Fig. 6b ). Whereas the estimated critical concentration for WT FtsZ was 0.09 μM, that of ΔCTL was increased to 0.57 μM and L14 to 0.97 μM, consistent with reduced longitudinal interactions ( Fig. 6b ). 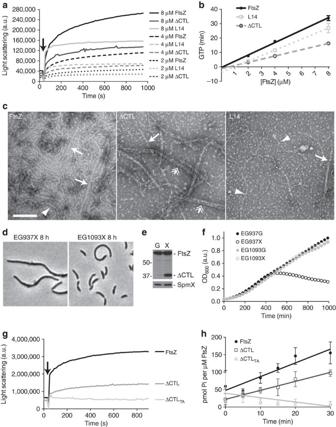Figure 6: ΔCTL must polymerize to cause bulging and lysis. (a) Right-angle light scattering over time by solutions containing purified 2, 4 or 8 μM WT FtsZ, ΔCTL or L14. Arrow indicates addition of GTP to induce polymerization. Curves are averages of three experiments. (b) GTPase activity of FtsZ variants fromaas a function of protein concentration. Averages±s.d. from three replicates are plotted with linear curve fits. Extrapolatedx-intercepts represent estimated critical concentration. (c) Negative stain electron micrographs of the indicated FtsZ variant at 8 μM in the presence of 2 mM GTP and 2.5 mM MgCl2. Arrows: paired protofilaments; double arrows: thick bundles; arrowheads: single protofilaments. Scale bar, 100 nm. (d) Phase contrast micrographs of EG937, bearing xylose-inducible ΔCTL, and EG1093, a spontaneous suppressor mutant of EG937 grown in xylose for 8 h. (e) Immunoblot of lysates from strain EG1093 grown in glucose or xylose for 24 h probed with FtsZ (top) or SpmX (bottom) antisera. Positions of molecular weight markers (kDa) are indicated (left). (f) Growth of EG937 and EG1093, with glucose (G) or xylose (X) added at time 0. (g) Right-angle light scattering over time by solutions containing purified 8 μM WT FtsZ, ΔCTL or ΔCTL T112A/A282T (ΔCTLTA). Arrow indicates addition of GTP to induce polymerization. Curves are averages of two experiments. (h) Inorganic phosphate liberated over time by 8-μM FtsZ variants fromf. Averages±s.d. from three replicates are plotted with linear curve fits. Figure 6: ΔCTL must polymerize to cause bulging and lysis. ( a ) Right-angle light scattering over time by solutions containing purified 2, 4 or 8 μM WT FtsZ, ΔCTL or L14. Arrow indicates addition of GTP to induce polymerization. Curves are averages of three experiments. ( b ) GTPase activity of FtsZ variants from a as a function of protein concentration. Averages±s.d. from three replicates are plotted with linear curve fits. Extrapolated x -intercepts represent estimated critical concentration. ( c ) Negative stain electron micrographs of the indicated FtsZ variant at 8 μM in the presence of 2 mM GTP and 2.5 mM MgCl 2 . Arrows: paired protofilaments; double arrows: thick bundles; arrowheads: single protofilaments. Scale bar, 100 nm. ( d ) Phase contrast micrographs of EG937, bearing xylose-inducible ΔCTL, and EG1093, a spontaneous suppressor mutant of EG937 grown in xylose for 8 h. ( e ) Immunoblot of lysates from strain EG1093 grown in glucose or xylose for 24 h probed with FtsZ (top) or SpmX (bottom) antisera. Positions of molecular weight markers (kDa) are indicated (left). ( f ) Growth of EG937 and EG1093, with glucose (G) or xylose (X) added at time 0. ( g ) Right-angle light scattering over time by solutions containing purified 8 μM WT FtsZ, ΔCTL or ΔCTL T112A/A282T (ΔCTL TA ). Arrow indicates addition of GTP to induce polymerization. Curves are averages of two experiments. ( h ) Inorganic phosphate liberated over time by 8-μM FtsZ variants from f . Averages±s.d. from three replicates are plotted with linear curve fits. Full size image We next examined the polymers formed by these CTL variants by negative stain TEM. At 4 μM protein concentration, few polymers were observed for ΔCTL or L14, indicating that they may be unstable. At 8 μM, we observed distinct polymer structures for each variant ( Fig. 6c ). While WT FtsZ assembled into single or paired protofilaments, L14 produced short, curved protofilaments and ΔCTL formed long, highly bundled polymers. These data demonstrate that the CTL contributes to efficient polymerization of FtsZ and that deletion of the CTL leads to increased protofilament bundling. To better understand the mechanism by which ΔCTL functions, we sought to identify suppressors of the bulging and lysis phenotype. To do this, we created a strain with WT ftsZ at the ftsZ locus and ΔCTL at the xylX locus and selected for clones that grew in the presence of xylose. One of the suppressors we isolated contained two point mutations in ΔCTL itself. This mutant grew equally well in the presence or absence of xylose and exhibited only mild filamentation in the presence of xylose ( Fig. 6d–f ). We confirmed that these are the only mutations required to suppress bulging and lysis by cloning ΔCTL with these point mutations into a vanillate-dependent FtsZ depletion background ( Supplementary Fig. 5c–e ). Interestingly, one of the mutations in the ΔCTL suppressor is in the tubulin signature motif required for GTP binding and hydrolysis (T112A) [30] , and the other is in the monomer–monomer interface (A283T) [31] ( Supplementary Figs 1 and 5b ). Each of these mutations is expected to impact polymerization. We tested the activity of the ΔCTL double mutant (ΔCTL TA ) and found that, as predicted, it does not polymerize and has no detectable GTPase activity ( Fig. 6g,h ). Thus, although ΔCTL has reduced polymerization activity as compared with WT FtsZ, our data suggest that it must polymerize to induce its toxic effects. ΔCTL induces specific changes to PG composition We next turned our attention to the cell envelope to ask how it is being perturbed by ΔCTL. We postulated that local breaches in the PG weakened the cell wall at sites of ΔCTL assembly, permitting bulging and lysis due to turgor pressure. A similar bulging filament phenotype has been reported in E. coli cells treated with penicillin [32] . Penicillin inhibits the penicillin-binding proteins (PBPs) that build the cell wall; therefore, we asked whether PG synthesis is disrupted in cells producing ΔCTL. To answer this, we pulse-labelled cells with a fluorescent D-alanine derivative (HADA) that is incorporated into the lipid II PG precursor and can be used to image sites of new PG synthesis [33] , [34] . As expected, HADA labelling of cells producing WT FtsZ yielded midcell bands of fluorescence, consistent with the bulk of PG synthesis in C. crescentus occurring at midcell [10] ( Fig. 7a , top). Surprisingly, in cells producing ΔCTL we observed robust HADA labelling at bulges ( Fig. 7a , bottom). However, the pattern of insertion over time was irregular for ΔCTL ( Supplementary Fig. 6 ), perhaps reflecting altered Z-ring organization or the incipient effects of membrane bulging through holes in the cell wall. From this we conclude that PG synthesis occurs at sites of ΔCTL assembly at least up to the step of transglycosylation, based on the mechanism of HADA incorporation. 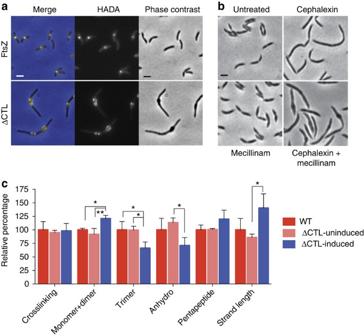Figure 7: Peptidoglycan crosslinking and glycan strand length are altered in cells producing ΔCTL. (a) Fluorescence (HADA) and phase contrast micrographs of strain EG852 grown with vanillate and glucose (top, FtsZ) or xylose (bottom, ΔCTL) for 5 h, and then pulse-labelled with HADA for 5 min before imaging. Scale bar, 2 μm. (b) Phase contrast images ofC. crescentuslacking β-lactamase (LS107) that were untreated, or treated with cephalexin, mecillinam or both for 6 h. Scale bar, 2 μm. (c) Relative abundance of total muropeptide crosslinking, the indicated crosslinked species, anhydroglycan ends, pentapeptides and glycan strand length of sacculi isolated from WTC. crescentus, or from EG852 grown in vanillate and glucose (ΔCTL-uninduced) or in xylose (ΔCTL-induced) for 5 h before sacculus preparation. Muropeptides were isolated and analysed in triplicate for each sample. Values are expressed as a percentage of the average WT value for each feature. Average+s.d. are presented.n=3 each. *P<0.05, **P<0.01 using one-way analysis of variance with Tukey’s multiple comparison post-test. Figure 7: Peptidoglycan crosslinking and glycan strand length are altered in cells producing ΔCTL. ( a ) Fluorescence (HADA) and phase contrast micrographs of strain EG852 grown with vanillate and glucose (top, FtsZ) or xylose (bottom, ΔCTL) for 5 h, and then pulse-labelled with HADA for 5 min before imaging. Scale bar, 2 μm. ( b ) Phase contrast images of C. crescentus lacking β-lactamase (LS107) that were untreated, or treated with cephalexin, mecillinam or both for 6 h. Scale bar, 2 μm. ( c ) Relative abundance of total muropeptide crosslinking, the indicated crosslinked species, anhydroglycan ends, pentapeptides and glycan strand length of sacculi isolated from WT C. crescentus , or from EG852 grown in vanillate and glucose (ΔCTL-uninduced) or in xylose (ΔCTL-induced) for 5 h before sacculus preparation. Muropeptides were isolated and analysed in triplicate for each sample. Values are expressed as a percentage of the average WT value for each feature. Average+s.d. are presented. n =3 each. * P <0.05, ** P <0.01 using one-way analysis of variance with Tukey’s multiple comparison post-test. Full size image Penicillin targets numerous PBPs, including transpeptidases and bifunctional enzymes. Using more specific inhibitors, it was reported that to invoke the bulging filament phenotype in E. coli , the division-specific transpeptidase, PBP3/FtsI, must be inhibited together with either the elongation-specific transpeptidase, PBP2 (ref. 35 ), or the lytic transglycosylase, Slt70 (refs 36 , 37 ), an enzyme that shortens glycan strands. We were able to recapitulate a bulging filament phenotype by treating C. crescentus cells lacking the β-lactamase gene with both cephalexin (a PBP3 inhibitor) and mecillinam (a PBP2 inhibitor; Fig. 7b ). On the basis of these data, we hypothesized that ΔCTL-mediated bulging and lysis results from reduced transpeptidation (crosslinking) and/or increased glycan strand length. To directly examine the changes to the PG induced by ΔCTL, we performed ultraperformance liquid chromatography (UPLC) analysis of muropeptides prepared from PG isolated from WT cells, or from the ΔCTL -expressing strain in the absence or presence of xylose ( Supplementary Fig. 7 ). Total muropeptide crosslinking was similar in the three samples ( Fig. 7c ). However, we observed an ∼ 30% decrease in the abundance of trimers (higher-order crosslinked species) in cells producing ΔCTL and a concomitant increase in the combined percentage of monomers and dimers. Our data and previous studies of C. crescentus PG [38] , [39] show that WT cells have shorter glycan strands than organisms such as E. coli , manifesting larger anhydro peaks representing the ends of glycan strands that allow for detection of increases in glycan strand length with greater fidelity. On ΔCTL expression, we detected an ∼ 50% increase in glycan strand length ( Fig. 7c ). These findings indicate that, consistent with the phenotypic similarity to chemical inhibition of PBP3 and PBP2 or Slt70, production of ΔCTL causes a decrease in higher-order transpeptidation and an increase in glycan strand length relative to cells producing WT FtsZ. The changes we observed in our muropeptide analysis may under-represent the extent of changes to the PG at the bulges, since the analysis aggregates PG composition from the entire cell and the ΔCTL-induced changes are likely to be highly localized. Midcell proteins are recruited to ΔCTL-mediated bulges The mechanisms by which cytoskeletal proteins such as FtsZ regulate cell wall metabolism are mostly unclear. One model posits that FtsZ serves only as a localization signal, bringing PG enzymes and their regulators to the appropriate location to carry out their functions. In C. crescentus , a number of proteins implicated in cell wall metabolism are sequentially enriched at midcell [9] . We hypothesized that in ΔCTL-producing cells, one or more of these factors might not be recruited to sites of FtsZ assembly, leading to alterations in PG metabolism. To test this, we examined the localization of ZBPs (ZapA, FzlA and FzlC), early recruits to midcell implicated in PG metabolism (MurG and DipM), and late divisome proteins involved in PG metabolism (PBP3/FtsI, FtsW and FtsN) in cells producing ΔCTL. Surprisingly, for each fluorescent protein fusion, we observed enrichment at ΔCTL-mediated bulges ( Fig. 8a,b , Supplementary Fig. 8a–f ). In addition, we performed in vitro co-sedimentation assays for MipZ and FzlA, two essential binding partners of FtsZ in C. crescentus . We observed similar levels of co-sedimentation of each with FtsZ and ΔCTL ( Supplementary Fig. 8g ). We conclude that the CTL is dispensable for binding of FtsZ to these essential partners and that midcell proteins are enriched at sites of Z-ring assembly in the presence of ΔCTL. This points to a mode of regulation of PG metabolism by FtsZ that is in addition to its ability to recruit proteins to midcell. 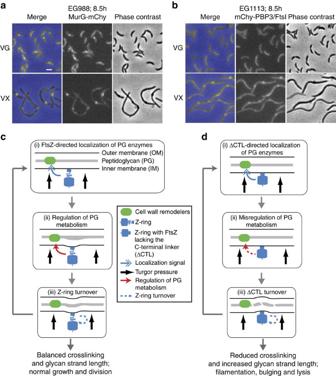Figure 8: PG enzymes are recruited to sites of ΔCTL assembly. (a,b) Fluorescence, phase contrast and merged images demonstrating localization of fluorescent fusions to divisome proteins in cells producing ΔCTL. MurG-mCherry and mCherry-FtsI were produced on vanillate induction in the EG937 background. Cells were grown in the presence of glucose or xylose for 8.5 h before imaging. Vanillate was added 2 h before imaging to induce expression of the fluorescent fusion. (c) Graphical representation of the role of FtsZ in promoting PG remodelling inC. crescentus. (i) Once established at the incipient division site, the Z-ring promotes local assembly of the divisome, including PG enzymes and their regulators. (ii) We propose that, in addition to recruiting PG enzymes to midcell, the Z-ring initiates a signal that regulates their activity, allowing appropriate re-shaping and invagination of the cell envelope. (iii) The Z-ring turns over, making constriction an iterative process. (d) When ΔCTL is produced, midcell proteins are still recruited (i), but their activities are misregulated (ii), leading to reduced PG crosslinking, increased glycan strand length, envelope bulging and cell lysis (iii). Figure 8: PG enzymes are recruited to sites of ΔCTL assembly. ( a , b ) Fluorescence, phase contrast and merged images demonstrating localization of fluorescent fusions to divisome proteins in cells producing ΔCTL. MurG-mCherry and mCherry-FtsI were produced on vanillate induction in the EG937 background. Cells were grown in the presence of glucose or xylose for 8.5 h before imaging. Vanillate was added 2 h before imaging to induce expression of the fluorescent fusion. ( c ) Graphical representation of the role of FtsZ in promoting PG remodelling in C. crescentus . (i) Once established at the incipient division site, the Z-ring promotes local assembly of the divisome, including PG enzymes and their regulators. (ii) We propose that, in addition to recruiting PG enzymes to midcell, the Z-ring initiates a signal that regulates their activity, allowing appropriate re-shaping and invagination of the cell envelope. (iii) The Z-ring turns over, making constriction an iterative process. ( d ) When ΔCTL is produced, midcell proteins are still recruited (i), but their activities are misregulated (ii), leading to reduced PG crosslinking, increased glycan strand length, envelope bulging and cell lysis (iii). Full size image The bacterial actin MreB also plays an important role in regulating PG metabolism and is enriched at midcell for much of the cell cycle in C. crescentus [40] , [41] . We therefore asked whether MreB midcell localization is required for the ΔCTL-induced PG misregulation we observe. To do this, we took advantage of previously described MreB mutants that are not recruited to midcell, but that support normal growth and division: MreB(D16G) [42] and MreB(Q26P) [7] . In both of these backgrounds, ΔCTL production induced filamentation, bulging and lysis in a manner similar to WT ( Supplementary Fig. 9 ). These data indicate that MreB is likely dispensable for the CTL-dependent mechanism by which FtsZ regulates PG metabolism. Cytoskeletal proteins in bacteria are required to specify and maintain cell shape, yet the mechanisms by which they regulate PG remodelling to achieve cell shape changes are largely undefined. Here we have provided evidence that the disordered CTL of FtsZ is required for the Z-ring to direct robust cell wall construction. We demonstrated that deletion of the CTL causes lethal defects in PG metabolism through a mechanism requiring ΔCTL polymerization and the membrane-anchoring CTC. In addition, we determined that, while the ability of ΔCTL to recruit proteins to midcell is intact, ΔCTL production leads to altered Z-ring structure and specific changes in PG composition. Our characterization of the ΔCTL variant has therefore allowed us to propose a PG-regulatory function for FtsZ that extends beyond its ability to simply recruit PG metabolic machinery to its site of assembly. In this study, we set out to characterize the role of the long CTLs found in α-proteobacterial FtsZs. Functional analysis of divergent CTLs and Cc CTL deletion variants indicated a sequence-dependent function for the CTL in C. crescentus ( Figs 1 and 2 , Supplementary Fig. 2 ). In addition to having notably long CTLs, α-proteobacteria also encode several ZBPs that are conserved only in this group [43] , [44] , [45] . We initially hypothesized that the CTL might act as a binding platform for one or more essential, α-proteobacterial-specific ZBPs. This does not appear to be the case, however, at least for known ZBPs: MipZ and FzlA interact equally well with purified WT and ΔCTL FtsZ ( Supplementary Fig. 8g ). An alternative sequence-dependent function may be to regulate FtsZ protein stability [23] , [46] or otherwise affect FtsZ levels post-transcriptionally. FtsZ levels vary over the cell cycle in C. crescentus , being subject to both transcriptional and proteolytic regulation [23] , [47] . We observed reduced steady-state levels of some CTL variants when expressed from equivalent constructs, and found that Nt34 and Ct36 were degraded more rapidly than WT FtsZ ( Supplementary Fig. 2f ). These effects on protein stability may be encoded in the CTL primary sequence as ClpXP protease recognition sites, as was recently demonstrated for E. coli FtsZ [46] . However, we have not identified any such sequences within the Cc CTL. Using E. coli proteins in vitro, polymeric FtsZ was shown to be degraded more rapidly by ClpXP than monomeric FtsZ [48] . CTL-dependent effects on FtsZ turnover may therefore be mediated indirectly, by altering the monomer–polymer ratio of FtsZ. Effects of the CTL on FtsZ levels is likely only part of the story, however, as the Rp CTL variant was present at nearly WT levels, yet failed to support division. The sequence-dependent function of the C. crescentus CTL lies in contrast to observations from E. coli and B. subtilis , where nearly any disordered sequence similar in length to the native CTL was sufficient to support normal division [19] , [20] . In B. subtilis , however, the presence of a CTL was required to prevent cell lysis, and in E. coli , one CTL variant (Add64blk) caused a ‘bulging and lysis’ defect and an increase in filament bundling similar to what we observed with ΔCTL [19] , [20] . The morphological changes associated with ΔCTL production in C. crescentus drew our attention to this phenomenon and highlighted a likely role for the CTL in regulating PG metabolism ( Fig. 3 ). We posit that in C. crescentus the CTL is at least bifunctional: it fulfils a sequence-dependent function required for efficient division and a minimal-length-dependent role in preventing misregulation of PG remodelling. A length-dependent, sequence-independent role for the CTL in executing cytokinesis may also exist in C. crescentus : many of the Cc CTL deletion variants we tested, while viable, performed cytokinesis inefficiently ( Fig. 2 ). We hypothesize that the role of a minimal CTL in preventing cell lysis is conserved and, if so, explains the presence of a CTL of at least nine residues in all FtsZ homologues bearing a CTC [18] . The surprising consequences of ΔCTL production indicate misregulation of a subset of cell wall remodelling activities. This differs from complete loss of FtsZ function, wherein a Z-ring fails to form, PG metabolism becomes dispersed [10] and cells grow as smooth filaments until lysis occurs many hours later [49] . Our muropeptide analysis revealed distinct alteration of the sacculus in ΔCTL-producing cells: they had reduced higher-order crosslinking and increased glycan strand length relative to cells producing WT FtsZ ( Fig. 7c ). The phenotypic similarity of ΔCTL production to inhibition of PBP3 and PBP2 or Slt70 along with the known activities of these enzymes is consistent with the possibility that they are inhibited by ΔCTL. Interestingly, a previous study reported similar changes to the cell wall when they inhibited MreB for several hours, and then allowed cells to recover MreB function [39] . The authors postulated an increase in transglycosylation activity to explain the observed changes. Although the CTL-dependent effects we describe appear to be MreB-independent ( Supplementary Fig. 9 ), a local increase in transglycosylation, without a coordinated increase in transpeptidation, could similarly explain the altered PG chemistry we observe with ΔCTL production. The next challenge is to explain ΔCTL-induced changes to the cell wall mechanistically. One can rationalize loss of localized cell wall metabolism when Z-rings completely fail to form if FtsZ acts simply as a localization signal. However, in ΔCTL-producing cells, insertion of new PG material is still localized to sites of FtsZ assembly ( Fig. 7a ) and all proteins we examined that normally localize to midcell were enriched at ΔCTL-mediated bulges ( Fig. 8a,b , Supplementary Fig. 8 ). These data disfavour a model for FtsZ function involving simple protein recruitment, although we cannot rule out the possibility that changes in protein localization in ΔCTL-producing cells occur that are too subtle to resolve using conventional light microscopy and/or are complicated by the geometry of ΔCTL-expressing cells. It is possible that FtsZ regulates PG metabolism through a scaffolding function that is more complex than simply positioning PG enzymes and their regulators at midcell. For example, the Z-ring may regulate the precise molecular architecture, stoichiometry, sequential order and/or dynamics of assembly and disassembly of protein complexes required for PG metabolism at the division site. There are unsolved mysteries regarding assembly of proteins downstream of FtsZ that hint at biophysical regulation of cell wall metabolism. In C. crescentus , MurG, which catalyses the final step in PG precursor synthesis, and DipM, a protein involved in PG hydrolysis, localize to midcell immediately after assembly of the Z-ring in an FtsZ-dependent manner [9] , [10] , [50] , [51] , [52] . However, neither MurG nor DipM interacts directly with FtsZ, nor do they require any other early recruit to midcell for their localization [9] , [43] . In fact, DipM resides in the periplasm and requires its PG-binding domains for localization [50] , [52] , suggesting special characteristics of PG at sites of the FtsZ assembly that mediate DipM recruitment. In addition, a number of inner membrane proteins are excluded from sites of FtsZ assembly through an unknown mechanism [43] , [53] . These observations indicate that the Z-ring alters the biophysical characteristics of the membrane [54] , [55] and/or PG locally to drive protein recruitment or exclusion. A similar biophysical mechanism might be invoked to regulate the activity of cell wall enzymes: we hypothesize that FtsZ initiates a physical signal that leads to local activation of PG metabolism ( Fig. 8c ). Such a signal is likely transduced through the CTC to FtsA and other effectors before ultimately being received by PG enzymes. Membrane-associated FtsZ is capable of generating constrictive force on membranes in vitro [4] . However, whether this force is generated in vivo and, if so, how such force is used during growth and division are unknown. One possibility is that FtsZ-mediated force is the physical signal described above: force generated by the Z-ring would be transduced to the cell envelope and/or divisome proteins and used to mechanically regulate the activity of PG remodelling enzymes ( Fig. 8c ). The CTL has been proposed to behave as an entropic spring [20] that is expected to affect the mechanical properties of FtsZ. Moreover, we observed altered FtsZ architecture for ΔCTL in cells and in vitro . We hypothesize that reduction of the CTL below a minimal length alters the physical properties of the Z-ring, including its ability to generate or transduce force, in a manner that leads to misregulation of cell wall remodelling ( Fig. 8d ). The unique phenotype associated with ΔCTL production provides a valuable genetic tool for further delineation of the mechanisms underlying the regulation of cell shape by the bacterial cytoskeleton. Bacterial strains and growth conditions C. crescentus NA1000 strains were grown in peptone yeast extract (PYE) medium or in minimal M2 medium at 30 °C. Additives and antibiotics were used at the following concentrations in liquid (solid) media for C. crescentus : xylose 0.3 (0.2)%, glucose 0.2%, vanillate 0.5 (0.5) mM, myo-inositol 0.3%, gentamycin 1 (5) μg ml −1 , kanamycin 5 (25) μg ml −1 , spectinomycin 25 (100) μg ml −1 , streptomycin (5 μg ml −1 ), cephalexin 1 μg ml −1 and mecillinam 5 μg ml −1 . Before changes in induction conditions, cells were washed two to three times in plain media. Growth rate analyses were performed in 96-well plates with shaking at 30 °C using a Tecan Infinite 200 Pro plate reader. Strains and plasmids used in this study are listed in Supplementary Data 1 and 2 . Light microscopy and image analysis Cells were imaged during the log phase of growth after immobilization on 1% agarose pads. Light microscopy was performed on a Nikon Eclipse Ti inverted microscope equipped with a Nikon Plan Fluor × 100 (numeric aperture 1.30) oil Ph3 objective and Photometrics CoolSNAP HQ [2] cooled CCD (charge-coupled device) camera. Chroma filter cubes were used as follows: ET-EYFP for YFP and Venus, ET-ECFP for CFP, ET-EGFP for GFP, ET-dsRED for mCherry and ET-DAPI for HADA. Images were processed in Adobe Photoshop. Automated cell width analysis was performed using MicrobeTracker [56] . Algorithm 4 was used for determining cell outlines, with the following parameter changes: areaMin=150, areaMax=5,000 and wspringconst=0.1. Maximum cell width along the entire length of the cell for each cell in the population was determined from this analysis. In cells with bulges, the maximum cell width corresponds to the width of the largest bulge. Whole-cell TEM Five microlitres of cells were spotted on carbon-coated mesh copper grids (Electron Microscopy Sciences, Fort Washington, PA) and allowed to adhere for 15 min. Grids were rinsed with ddH 2 O and stained with 7.5% uranyl magnesium acetate for 5 min. The grids were rinsed in ddH 2 O five times and allowed to dry briefly before placing in a grid box. Grids were imaged the next day at 80 kV using a JEOL JEM 1010 transmission electron microscope equipped with a 4 k × 4 k Gatan CCD Ultrascan 4000 SP model 890 camera. Antibodies and immunoblotting Purified full-length C. crescentus FtsZ was used to immunize a rabbit for antibody production (Josman, LLC). Specificity for FtsZ was demonstrated by immunoblotting lysates from strains depleted of FtsZ and observing a reduction in the signal at the expected molecular weight of full-length C. crescentus FtsZ (predicted 54 kDa, runs at ∼ 65 kDa; for example, Supplementary Fig. 2c ) and by producing FtsZ variants and observing new bands at the expected molecular weight (for example, Supplementary Fig. 3 ). For immunoblotting against whole-cell lysates, cells were harvested in the log phase of growth and lysed in SDS–PAGE loading buffer by boiling for 5 min. SDS–PAGE and transfer of protein to nitrocellulose membrane were performed using standard procedures. FtsZ antiserum was used at 1:20,000 dilution. SpmX antiserum was used at 1:50,000 dilution [57] . Uncropped immunoblots are presented in Supplementary Fig. 3 . Protein stability assay Translation was inhibited by adding chloramphenicol (30 μg ml −1 ) to strains expressing WT FtsZ or linker variants as the only copy of FtsZ. Cells were harvested every 20 min for 2 h, and lysates from each time point (equivalent total OD units loaded for each) were subjected to immunoblotting with FtsZ antiserum. Horseradish peroxidase-conjugated secondary antibody and ECL substrate were used for detection. Signal was detected using an ImageQuant LAS4000 mini chemiluminescence imaging system (GE Healthcare Life Sciences, Piscataway, NJ) and quantified with the ImageQuant TL software. Protein half-life was calculated by plotting the relative concentration (normalized to amount of FtsZ or FtsZ variant at time 0) against time and fitting a one-phase decay curve using the Graphpad Prism software (Graphpad Software Inc., La Jolla, CA). Protein purification FtsZ, FtsZ variants, His 6 -FzlA and His 6 -MipZ were overproduced and purified as described previously [43] with slight modifications. To purifiy FtsZ, Rosetta (DE3) pLysS E. coli cells bearing plasmid pMT219 were grown at 37 °C to OD 600 of 0.8–1.0 before induction with 0.5 mM isopropylthiogalactoside (IPTG) for 3–4 h. Cells were harvested by centrifugation at 6,000 g for 10 min at 4 °C, resuspended in 30 ml Buffer QA (50 mM Tris-HCl pH 8.0, 50 mM KCl, 1 mM EDTA, 1 mM β-mercaptoethanol and 10% glycerol) per litre of culture, snap-frozen in liquid nitrogen and stored at −80 °C until purification. Cell suspensions were thawed, one Mini Complete Protease Inhibitor tablet was added per 30 ml (Roche), lysozyme was added to 1 mg ml −1 , phenylmethyl sulphonyl fluoride (PMSF) was added to 2 mM and DNAse I (New England Biolabs) was added to 2 units ml −1 final concentrations. Cell suspensions were incubated for 30–60 min at room temperature, sonicated and centrifuged at 15,000 g for 30 min at 4 °C. Supernatant was filtered and loaded on two HiTrap Q HP 5 ml columns (GE Life Sciences) joined in tandem and equilibrated in Buffer QA. Protein was eluted using a linear KCl gradient from 50 to 500 mM over 20 column volumes. Peak fractions containing FtsZ were combined and ammonium sulfate was added to 20% saturation. Ammonium sulfate precipitate was recovered with centrifugation at 10,000 g for 10 min at 4 °C. After resting overnight on ice, precipitates were resuspended in FtsZ Storage Buffer (50 mM HEPES-KOH pH 7.2, 50 mM KCl, 0.1 mM EDTA, 1 mM β-mercaptoethanol and 10% glycerol) and consecutively applied to a Superdex 200 10/300 GL column (GE Life Sciences) in FtsZ Storage Buffer. Peak fractions were combined, concentrated if necessary, snap-frozen in liquid nitrogen and stored at −80 °C. ΔCTL, L14 and ΔCTL TA FtsZ variants were overproduced from plasmids pEG681, pEG723 and pEG886, respectively, in Rosetta (DE3) pLysS E. coli as for FtsZ and purified following the same procedure used for FtsZ. The only exceptions were that ΔCTL precipitated at 30% ammonium sulfate and ΔCTL TA precipitated at 40% ammonium sulfate. To purify His 6 -MipZ, Rosetta (DE3) pLysS E. coli cells bearing plasmid pMT183 were grown at 37 °C to OD 600 of 0.6 before induction with 0.5 mM IPTG for 3.25 h. Cells were harvested by centrifugation at 6,000 g for 10 min at 4 °C, washed in PBS, snap-frozen in liquid nitrogen and stored at −80 °C until purification. Cells were thawed and resuspended in Ni lysis buffer (50 mM Tris-HCl pH 8.0, 300 mM NaCl, 10 mM imidazole, 1 mM EDTA and 10% glycerol). One Mini Complete Protease Inhibitor tablet was added per 30 ml (Roche), PMSF was added to 2 mM and DNAse I (New England Biolabs) was added to 2 units ml −1 final concentrations. Cells were lysed by passage through a French Press twice at 15,000 psi and lysates were centrifuged at 15,000 g for 30 min at 4 °C. His 6 -MipZ was isolated by binding to Ni-NTA agarose (Qiagen), washed in Ni wash buffer (Ni lysis buffer with 20 mM imidazole) and eluted in Ni elution buffer (Ni lysis buffer with 300 mM imidazole). Peak fractions were concentrated and applied to a Superdex 200 10/300 GL column (GE Life Sciences) equilibrated in MipZ Storage Buffer (50 mM HEPES-NaOH pH 7.2, 50 mM NaCl, 0.1 mM EDTA, 1 mM β-mercaptoethanol and 10% glycerol). Peak fractions were pooled, concentrated, snap-frozen in liquid nitrogen and stored at −80 °C. To purifiy His 6 -FzlA, Rosetta (DE3) pLysS E. coli cells bearing plasmid pEG327 were grown at 30 °C to OD 600 of 0.5 before induction with 0.5 mM IPTG for 4 h. Cells were harvested by centrifugation at 6,000 g for 10 min at 4 °C, resuspended in FzlA lysis buffer (50 mM Tris-HCl pH 8.0, 300 mM NaCl, 20 mM imidazole and 10% glycerol), snap-frozen in liquid nitrogen and stored at −80 °C until purification. Cells were thawed and lysozyme was added to 1 mg ml −1 , one Mini Complete Protease Inhibitor tablet was added per 30 ml (Roche), MgCl 2 was added to 2.5 mM and DNAse I (New England Biolabs) was added to 2 units ml −1 final concentrations. Cells were incubated at room temperature for 45 min, sonicated and lysates were centrifuged at 15,000 g for 30 min at 4 °C. Lysate was filtered and applied to two 1-ml HisTrap FF columns joined in tandem (GE Life Sciences) and equilibrated in FzlA lysis buffer. Columns were washed in FzlA lysis buffer, and His 6 -FzlA was eluted in FzlA elution buffer (FzlA lysis buffer with 300 mM imidazole). Peak fractions were combined, dialysed into FzlA Storage Buffer (50 mM Tris-HCl pH 8.0, 300 mM NaCl and 5% glycerol), snap-frozen in liquid nitrogen and stored at −80 °C. FtsZ activity assays FtsZ activity assays were performed in HEK50 buffer (50 mM HEPES-KOH pH 7.2, 50 mM KCl and 0.1 mM EDTA). MgCl 2 was used at 2.5 mM and GTP was used at 2 mM. Light scattering was monitored using a Fluoromax-3 spectrofluorometer (Jobin Yvon Inc.) with 350-nm excitation and emission wavelengths and 2-nm slits. GTPase activity was assayed using the SensoLyte MG Phosphate Assay Kit (AnaSpec) following the manufacturer’s protocol. The GraphPad Prism software was used to fit curves and determine GTPase rates. For pelleting and co-sedimentation assays, FtsZ was polymerized for 15 min at room temperature, with additional proteins when indicated. Reactions were subjected to centrifugation at 250,000 g for 15 min at 25 °C, after which supernatant and pellet fractions were collected. Critical concentration was estimated as the x -intercept in GTPase activity versus protein concentration plots. For visualization of protofilaments using TEM, 8 μM of purified protein was polymerized in HEK50 buffer with 2.5 mM MgCl 2 and 2 mM GTP for ∼ 15 min, spotted on glow-discharged carbon-coated mesh copper grids (Electron Microscopy Sciences, Hatfield, PA), dried after 2 min and stained with 0.75% uranyl formate for 2 min. The grids were dried once again and the staining was repeated. The grids were completely dried and imaged using a Philips/FEI BioTwin CM120 TEM equipped with an AMT XR80 8 megapixel CCD camera (AMT Imaging, USA). HADA labelling Strain EG852 was washed twice in PYE and resuspended in PYE with either vanillate and glucose (to induce WT ftsZ ) or xylose (to induce ΔCTL ). Cells were grown for 5 h at 30 °C with shaking, HADA [34] was added to a final concentration of 0.41 mM and cells were returned to the shaker for 5 min. Cells were removed, washed twice in PBS, resuspended in ice-cold 70% ethanol and incubated on ice for 20 min. Cells were pelleted, resuspended in PBS and imaged. For pulse-chase labelling, following 5 min incubation with HADA, cells were washed twice in PYE, resuspended in PYE with supplements and returned to the incubator. Cells were withdrawn at time zero or indicated times and processed for imaging as above. Muropeptide analysis UPLC samples were prepared as described previously [58] , with modifications. Log phase cultures of C. crescentus EG852 and EG864 were washed in PYE and diluted 1:10 in 500 ml plain PYE (EG864), PYE with vanillate plus glucose (EG852 ΔCTL-uninduced) or PYE with xylose (EG852 ΔCTL-induced). Cultures were grown for 5 h at 30 °C to an OD 600 of 0.3, and then centrifuged at 6,000 g for 10 min at 4 °C. The resulting pellets were resuspended in 3 ml ice-cold water. Cell suspensions were then lysed by boiling in 6% SDS for 30 min and allowed to cool to room temperature. Lysed cell suspensions were ultracentrifuged at 400,000 g and pelleted sacculi were digested with muramidase into muropeptides. Samples were pH-adjusted, injected on a Waters H Class UPLC system equipped with a BEH C18 1.7-μm column (Waters, MA, USA) and eluted with sodium phosphate buffers. Peaks were quantified and identified as particular muropeptide species from their elution times based on ref. 39 , from which the crosslinking density and strand length were calculated [59] . How to cite this article: Sundararajan, K. et al. The bacterial tubulin FtsZ requires its intrinsically disordered linker to direct robust cell wall construction. Nat. Commun. 6:7281 doi: 10.1038/ncomms8281 (2015).